Rapid calcium-dependent activation of Aurora-A kinase Oncogenic hyperactivation of the mitotic kinase Aurora-A (AurA) in cancer is associated with genomic instability. Increasing evidence indicates that AurA also regulates critical processes in normal interphase cells, but the source of such activity has been obscure. We report here that multiple stimuli causing release of Ca 2+ from intracellular endoplasmic reticulum stores rapidly and transiently activate AurA, without requirement for second messengers. This activation is mediated by direct Ca 2+ -dependent calmodulin (CaM) binding to multiple motifs on AurA. On the basis of structure–function analysis and molecular modelling, we map two primary regions of CaM-AurA interaction to unfolded sequences in the AurA N- and C-termini. This unexpected mechanism for AurA activation provides a new context for evaluating the function of AurA and its inhibitors in normal and cancerous cells. The Aurora-A (AurA) kinase is a member of the evolutionarily conserved Ipl family of kinases (reviewed in Marumoto et al . [1] ). AurA is most abundant at the centrosome in G2 to M phase [2] , and in studies performed in mammals and model organisms including Drosophila , AurA has been shown to be activated at mitotic entry, performing critical functions in regulating entry into and passage through mitosis [1] , [3] . Activation of AurA at mitosis is supported by a complex set of interactions between the protein and a number of partners, including Ajuba [4] , Pak [5] , Bora [6] , TPX2 [7] , PPI2 [8] and NEDD9 [9] . These interactions typically occur at the centrosome, with the partner proteins supporting AurA localization and stability, and inducing allosteric changes that contribute to AurA activation. Because of the complex nature of the interactions, the exact mechanism timing the abrupt AurA activation at the mitotic boundary has not been well resolved. In the past several years, AurA has attracted increasing attention because it has been found to be overexpressed and hyperactivated in a high percentage of tumours arising in breast, colon, ovary and other tissues [10] , [11] , [12] , [13] , [14] . Abnormally high AurA activity is oncogenic in various cell line models and is associated with defective cytokinesis and aneuploidy [15] , [16] , [17] , [18] . AurA is now being actively exploited as a target for development of new anti-cancer agents (reviewed in Andrews [19] ) on the basis of this known role as a mitotic regulator. Interestingly, the overexpressed AurA associated with cancer cells has a number of activities that are not specific to function in a mitotic compartment. For example, AurA directly phosphorylates and regulates the activity of the RalA GTPase, an EGFR/Ras effector important in many cancers [20] , with this activity observed in interphase cells. AurA is not typically mutationally activated in cancer, making the mechanism of its activation in interphase cells somewhat elusive. Intriguingly, a number of studies have emerged in recent years to challenge the idea that AurA is solely a mitotic kinase even in normal cells. Serum induces AurA activation at the basal body of the cell cilium in non-cycling G0/G1-phase mammalian cells, causing AurA-dependent ciliary resorption [21] , and hence indirectly impacting the functionality of the cilia-dependent and cancer-relevant Hedgehog signalling cascades [22] . AurA also has been reported to regulate microtubule dynamics in interphase cells [23] , and has been shown to be abundantly expressed in some human adult non-cycling tissues such as kidney [24] . All these studies strongly imply a non-mitotic activity for AurA, and indeed, a distant ortholog of AurA in the green algae Chlamydomonas regulates both resorption and excision of the flagella (a structure analogous to the mammalian cilium) in response to altered ionic conditions or cues for mating [25] , again suggesting important non-mitotic roles for AurA, although across a great evolutionary distance. However, to date, little effort has been made to investigate the non-mitotic activation of AurA in either normal cells or tumours, and mechanistic insight into factors governing such activation is essentially absent. Our previous work demonstrating that AurA activation occurs before ciliary resorption in interphase cells [21] was based on studies in Chlamydomonas , which implicated an AurA ortholog, CALK, as important for resorption of flagella in that organism [25] . Stimuli that lead to loss of flagella in Chlamydomonas include mating response to pheromone and transient ionic shock [25] . Recent studies in Chlamydomonas have also suggested increasing intraflagellar calcium concentrations during the mating response [26] , shortly before the activation of the CALK kinase. Independently, a study of the Chlamydomonas flagellar excision process emphasized the importance of rapid spatiotemporal patterning of calcium ion distribution as a critical mediating signal [27] . Interestingly, a recent study of oocyte maturation in Xenopus indicated that inhibition of Ca 2+ signalling led to eventual failure to accumulate and activate AurA [28] , although no direct connection was investigated. Cumulatively, these studies led us to hypothesize that AurA might be a direct target of cellular calcium signalling in mammals. Our work presented here demonstrates that elevated cytoplasmic calcium signals are transmitted rapidly and transiently through calmodulin (CaM) to activate AurA. This activation involves direct CaM binding to two sites in the unstructured regions of AurA, and induced by multiple inducers of calcium release from intracellular stores in the endoplasmic reticulum (ER). These results provide the first clear mechanism for AurA activation in non-mitotic cells and potential insight into the timing of activation of AurA at mitosis. ER release of Ca 2+ rapidly and transiently activates AurA Rapid and transient Ca 2+ channel activity is stimulated by treatment of kidney cells with the peptide hormone and anti-diuretic arginine vasopressin (AVP) [29] , [30] . AVP signals through the AVPR1 receptor to initiate InsP3 and other second-messenger cascades that initiate Ca 2+ release from the ER. The AVPR1 receptor is well expressed in the renal cell lines HK-2 and HEK293 ( Fig. 1a ). To assess whether activation of AurA occurred in this physiological context, we treated the HK-2 proximal tubule-derived human kidney cell line with AVP, and used immunofluorescence with antibody directed to T 288 (auto-phosphorylated)-AurA to measure AurA activation ( Fig. 1b ). Strikingly, T 288 -phospho AurA at centrosomes increased threefold within 5 s of AVP treatment, returning to basal levels after ~2 min ( Fig. 1c ), whereas total AurA levels were not affected ( Fig. 1d ). AurA activation might be mediated by Ca 2+ influx from outside the cell, or by Ca 2+ released from internal ER stores. Using AurA-transfected HEK293 cells, we found an equivalent degree of AurA activation after AVP treatment of cells cultured in medium with and without Ca 2+ ( Fig. 1e ). To confirm that activation was not specific to the AVP-initiating stimulus, we also treated these cells grown in Ca 2+ -free medium with histamine, an InsP3 generating agonist that triggers activation of ER-associated calcium ion channels such as the IP3 receptor [31] . Again T 288 -AurA appeared rapidly after stimulation ( Fig. 1f ). 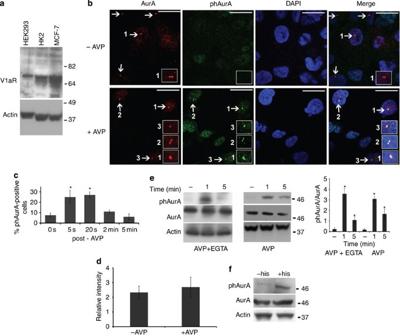Figure 1: Calcium release rapidly induces AurA auto-phosphorylation. (a) Western blot assay confirming expression of the AVPR1 receptor in cell lines used in this study. MCF7 were used as a positive control for AVPR1 expression, based on Northet al.60. (b) Immunofluorescence of HK-2 cells 30 s after stimulation with 100 nM arginine vasopressin (+AVP) versus control untreated cells (−AVP). Cells were visualized with antibodies to AurA (red) and T288-phospho-AurA (phAurA, green) and DAPI (blue), as indicated; scale bar, 20 μm. Insets show magnification of indicated centrosomes. (c) Analysis of data frombquantifies phAurA-positive cells at times after stimulation. (d) Analysis of data frombquantifies relative intensity of AurA in cells within 20 s after stimulation with AVP. (e) Western blot analysis of AVP-treated HEK293 cells overexpressing AurA in the presence or absence of extracellular Ca2+chelator (5 mM EGTA) (f) Western blot analysis of phAurA in HEK293 cells transfected with an AurA-expressing plasmid 1–2 min after stimulation with 10 μM histamine. For each SDS–PAGE, β-actin is used as a loading control and molecular weight is indicated in kDa. Forcandd, an average of 150 cells were counted. (c,d,e)N=3 with error bars indicating the standard error. *P<0.05. Figure 1: Calcium release rapidly induces AurA auto-phosphorylation. ( a ) Western blot assay confirming expression of the AVPR1 receptor in cell lines used in this study. MCF7 were used as a positive control for AVPR1 expression, based on North et al . [60] . ( b ) Immunofluorescence of HK-2 cells 30 s after stimulation with 100 nM arginine vasopressin (+AVP) versus control untreated cells (−AVP). Cells were visualized with antibodies to AurA (red) and T 288 -phospho-AurA (phAurA, green) and DAPI (blue), as indicated; scale bar, 20 μm. Insets show magnification of indicated centrosomes. ( c ) Analysis of data from b quantifies phAurA-positive cells at times after stimulation. ( d ) Analysis of data from b quantifies relative intensity of AurA in cells within 20 s after stimulation with AVP. ( e ) Western blot analysis of AVP-treated HEK293 cells overexpressing AurA in the presence or absence of extracellular Ca 2+ chelator (5 mM EGTA) ( f ) Western blot analysis of phAurA in HEK293 cells transfected with an AurA-expressing plasmid 1–2 min after stimulation with 10 μM histamine. For each SDS–PAGE, β-actin is used as a loading control and molecular weight is indicated in kDa. For c and d , an average of 150 cells were counted. ( c , d , e ) N =3 with error bars indicating the standard error. * P <0.05. Full size image The fact that rapid AurA activation occurred after stimulation of cells grown without extracellular Ca 2+ implied that the elevated cytoplasmic Ca 2+ levels resulting from ER release might regulate AurA activation without intrinsic requirement for second messengers transmitting signals from membrane-localized receptors. To further assess this mechanism, we treated AurA-transfected HEK293 cells with the Ca 2+ uptake inhibitor thapsigargin, which blocks the recycling of cytoplasmic Ca 2+ into ER stores [32] , thus increasing cytoplasmic Ca 2+ levels without the involvement of upstream activators. Thapsigargin treatment caused a rapid (<1 min) increase in levels of activated T 288 -AurA, and increased the in vitro kinase activity of immunoprecipitated AurA against defined substrates ( Fig. 2a,b ). 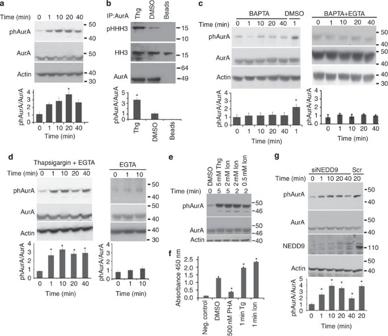Figure 2: Intracellular calcium release is sufficient for AurA activation. (a) HEK293 cells overexpressing AurA were incubated with 5 μM thapsigargin for the indicated periods of time, and then cell lysates were analysed by western blot. Graph shown below indicates ratio of phAurA to total AurA. (b) AurA immunoprecipitation andin vitrokinase assay, after thapsigargin treatment. HEK293 cells overexpressing AurA were treated with 5 μM thapsigargin or control dimethylsulpfoxide (DMSO) for 5 min, AurA was immunoprecipitated and incubated with histone H3 substrate in anin vitrokinase assay. phHH3, antibody to phosphorylated histone H3. *P<0.05. (c) Left, an experiment similar to that shown ina, except that it is performed in the presence of 50 μM BAPTA-AM or control DMSO. Right, HEK293 cells overexpressing AurA were incubated with 20 μM BAPTA-AM (30 min) plus 7.5 mM EGTA (2 min) before the addition of 5 μM thapsigargin for the indicated periods of time, with analysis as fora. (d) An experiment similar to that shown ina, except that it is performed in the presence of 5 mM EGTA alone for the indicated periods of time (right panel) or in the presence of 5 mM EGTA (2 min) before the addition of 5 μM thapsigargin. (e) HEK293 cells overexpressing AurA were incubated with 5 μM thapsigargin and indicated concentration of ionomycin for the indicated periods of time, and then cell lysates were analysed by western blot using indicated antibodies. (f) HK2 cells were treated with DMSO, 5 μM thapsigargin (Tg) or 0.5 μM ionomycin (Ion), and then T288-phAurA levels were analysed by enzyme-linked immunosorbent assay (ELISA), based on A450 nm. To confirm the specificity of ELISA signal, a parallel group of HK2 cells were pre-treated with the AurA inhibitor PHA680632 (PHA) at 500 nM concentration. *P=0.05. Lysis buffer was used as a negative control. (g) AurA-overexpressing HEK293 cells were transfected with siRNA-depleting NEDD9 (siNEDD9) or scrambled control siRNA (scr), and then were incubated with 5-μm thapsigargin and processed as ina. For this and subsequent SDS–PAGE analyses, each experiment was performed three times independently, with error bars indicating the standard error. *P<0.05. Figure 2: Intracellular calcium release is sufficient for AurA activation. ( a ) HEK293 cells overexpressing AurA were incubated with 5 μM thapsigargin for the indicated periods of time, and then cell lysates were analysed by western blot. Graph shown below indicates ratio of phAurA to total AurA. ( b ) AurA immunoprecipitation and in vitro kinase assay, after thapsigargin treatment. HEK293 cells overexpressing AurA were treated with 5 μM thapsigargin or control dimethylsulpfoxide (DMSO) for 5 min, AurA was immunoprecipitated and incubated with histone H3 substrate in an in vitro kinase assay. phHH3, antibody to phosphorylated histone H3. * P <0.05. ( c ) Left, an experiment similar to that shown in a , except that it is performed in the presence of 50 μM BAPTA-AM or control DMSO. Right, HEK293 cells overexpressing AurA were incubated with 20 μM BAPTA-AM (30 min) plus 7.5 mM EGTA (2 min) before the addition of 5 μM thapsigargin for the indicated periods of time, with analysis as for a . ( d ) An experiment similar to that shown in a , except that it is performed in the presence of 5 mM EGTA alone for the indicated periods of time (right panel) or in the presence of 5 mM EGTA (2 min) before the addition of 5 μM thapsigargin. ( e ) HEK293 cells overexpressing AurA were incubated with 5 μM thapsigargin and indicated concentration of ionomycin for the indicated periods of time, and then cell lysates were analysed by western blot using indicated antibodies. ( f ) HK2 cells were treated with DMSO, 5 μM thapsigargin (Tg) or 0.5 μM ionomycin (Ion), and then T 288 -phAurA levels were analysed by enzyme-linked immunosorbent assay (ELISA), based on A 450 nm . To confirm the specificity of ELISA signal, a parallel group of HK2 cells were pre-treated with the AurA inhibitor PHA680632 (PHA) at 500 nM concentration. * P =0.05. Lysis buffer was used as a negative control. ( g ) AurA-overexpressing HEK293 cells were transfected with siRNA-depleting NEDD9 (siNEDD9) or scrambled control siRNA (scr), and then were incubated with 5-μm thapsigargin and processed as in a . For this and subsequent SDS–PAGE analyses, each experiment was performed three times independently, with error bars indicating the standard error. * P <0.05. Full size image As another test, the BAPTA-AM Ca 2+ ion chelator blocks Ca 2+ -mediated signalling pathway activation [33] ; BAPTA-AM used alone or at low concentration in combination with EGTA completely blocked thapsigargin-induced T 288 -AurA auto-phosphorylation ( Fig. 2c ). In the absence of BAPTA-AM, EGTA (which chelates only extracellular Ca 2+ ) had no effect either used alone or in conjunction with thapsigargin ( Fig. 2d ). In addition, treatment with the Ca 2+ -selective ionophore, ionomycin, which directly triggers Ca 2+ release, similarly induced transient activation of AurA with similar kinetics ( Fig. 2e ). Further, a small molecule inhibitor of AurA, PHA680632 [34] , blocked thapsigargin- or ionomycin-induced AurA auto-phosphorylation ( Fig. 2f ). The AurA partner protein, NEDD9, has been shown to be important for AurA activation in mitosis and in ciliary resorption [9] , [21] , and been shown to be rapidly tyrosine phosphorylated (associated with more efficient function as an activator for some NEDD9 partner proteins) after Ca 2+ release in osteoclasts [35] , [36] . However, in cells transfected with small interfering RNA-depleting NEDD9, thapsigargin induced comparable AurA phosphorylation to that in control transfected cells ( Fig. 2g ). These data indicated that calcium-activated AurA phosphorylation is independent from NEDD9 activity, causing us to investigate other activation mechanisms. Ca 2+ induces CaM to bind and activate AurA Increased cytoplasmic Ca 2+ might induce AurA activation by direct binding or by inducing conformational changes in AurA based on AurA binding to a Ca 2+ effector such as CaM. In an in vitro kinase assay, titration of Ca 2+ into the reaction did not affect AurA auto-phosphorylation or activity towards substrates such as histone H3 ( Fig. 3a ). However, addition of Ca 2+ with CaM strongly induced AurA auto-phosphorylation, as well as AurA phosphorylation of multiple canonical substrates including histone H3, MBP and NEDD9 ( Fig. 3a–c ). In addition, the AurA inhibitor PHA680632 also blocked CaM-induced phosphorylation ( Fig. 3c ). 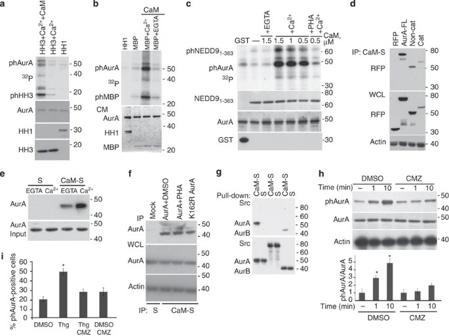Figure 3: CaM binds and activates AurA. (a)In vitrokinase assay using recombinant AurA, with the addition of Ca2+or CaM as indicated, with histone H3 (HH3)-positive and histone H1 (HH1)-negative control.32P-γ-ATP signal at ~55 kDa indicates AurA auto-phosphorylation. Similar activation of AurA was obtained with concentrations of Ca2+as low as 0.5 μM. (b)In vitrokinase assay using recombinant AurA, with the addition of CaM and Ca2+as indicated, with MBP used as AurA substrate and histone H1 as negative control. (c)In vitrokinase assay shows that CaM activates AurA. Top,32P-γ-ATP signal at ~55 kDa indicates AurA auto-phosphorylation, and signal at ~55 kDa indicates phosphorylation of NEDD91-363substrate. Bottom, representation of all indicated proteins in the reaction mixture. The AurA inhibitor PHA680632 (PHA) was used at 1 μM. (d) CaM-Sepharose (CaM-S) was used for immunoprecipitation (IP) from whole cell lysates (WCL) transfected with plasmids expressing red fluorescent protein (RFP), AurA-RFP and RFP-fused N-terminal (non-cat) and C-terminal (cat, kinase domain) of AurA, followed by western blotting. (e) AurA pulldown with CaM-Sepharose is Ca2+dependent. Recombinant AurA plus 1mM CaCl2(Ca2+) or 1 mM EGTA was incubated with CaM-Sepharose (CaM-S) or control Sepharose (S). (f). Experiment is carried out as ine, except that AurA is incubated with dimethylsulpfoxide (DMSO) or the AurA kinase inhibitor, PHA-680632, or a kinase-dead mutant of AurA (K162R) is used for pulldown. (g) Experiment is carried out as ine, performed in the presence of 1 mM Ca2+. (h) Western blot of lysates from HEK293 cells overexpressing AurA were preincubated for 1 h with 10 μM of the CaM inhibitor calmidazolium (CMZ) or control DMSO, incubated with 5 μM thapsigargin. Graph indicates ratio of phAurA to total AurA, quantified from analysis of three blots; error bars show standard error; *P<0.05. (i) HK2 cells were preincubated for 1 h with 10 μM CMZ or DMSO, treated with 5-μm thapsigargin for 1 min and then analysed by immunofluorescence with antibodies to AurA and T288-phospho-AurA. An average of 150 cells were counted in each of three experiments, with error bars indicating the standard error. *P=0.00054. Figure 3: CaM binds and activates AurA. ( a ) In vitro kinase assay using recombinant AurA, with the addition of Ca 2+ or CaM as indicated, with histone H3 (HH3)-positive and histone H1 (HH1)-negative control. 32 P-γ-ATP signal at ~55 kDa indicates AurA auto-phosphorylation. Similar activation of AurA was obtained with concentrations of Ca 2+ as low as 0.5 μM. ( b ) In vitro kinase assay using recombinant AurA, with the addition of CaM and Ca 2+ as indicated, with MBP used as AurA substrate and histone H1 as negative control. ( c ) In vitro kinase assay shows that CaM activates AurA. Top, 32 P-γ-ATP signal at ~55 kDa indicates AurA auto-phosphorylation, and signal at ~55 kDa indicates phosphorylation of NEDD9 1-363 substrate. Bottom, representation of all indicated proteins in the reaction mixture. The AurA inhibitor PHA680632 (PHA) was used at 1 μM. ( d ) CaM-Sepharose (CaM-S) was used for immunoprecipitation (IP) from whole cell lysates (WCL) transfected with plasmids expressing red fluorescent protein (RFP), AurA-RFP and RFP-fused N-terminal (non-cat) and C-terminal (cat, kinase domain) of AurA, followed by western blotting. ( e ) AurA pulldown with CaM-Sepharose is Ca 2+ dependent. Recombinant AurA plus 1mM CaCl 2 (Ca 2+ ) or 1 mM EGTA was incubated with CaM-Sepharose (CaM-S) or control Sepharose (S). ( f ). Experiment is carried out as in e , except that AurA is incubated with dimethylsulpfoxide (DMSO) or the AurA kinase inhibitor, PHA-680632, or a kinase-dead mutant of AurA (K162R) is used for pulldown. ( g ) Experiment is carried out as in e , performed in the presence of 1 mM Ca 2+ . ( h ) Western blot of lysates from HEK293 cells overexpressing AurA were preincubated for 1 h with 10 μM of the CaM inhibitor calmidazolium (CMZ) or control DMSO, incubated with 5 μM thapsigargin. Graph indicates ratio of phAurA to total AurA, quantified from analysis of three blots; error bars show standard error; * P <0.05. ( i ) HK2 cells were preincubated for 1 h with 10 μM CMZ or DMSO, treated with 5-μm thapsigargin for 1 min and then analysed by immunofluorescence with antibodies to AurA and T 288 -phospho-AurA. An average of 150 cells were counted in each of three experiments, with error bars indicating the standard error. * P =0.00054. Full size image These results predicted direct AurA-CaM binding. This binding was confirmed both in vitro and in vivo ( Fig. 3d, e ), and was positively regulated by Ca 2+ ( Fig. 3e ). Treatment with PHA680632 had no effect on AurA-CaM binding ( Fig. 3f ), as would be expected based on defined PHA680632 interactions with a unique site in the hinge region of the AurA catalytic domain [37] . CaM pulldown was specific to AurA, as a much weaker pulldown was seen with the related Ipl kinase AurB and no pulldown was seen with an unrelated kinase, Src ( Fig. 3g ). Further, thapsigargin-induced activation of endogenous AurA in HK-2 cells and of transfected AurA in HEK293 cells was completely blocked by the CaM inhibitor calmidazolium ( Fig. 3h, i ). Using mass spectrometry, we determined that addition of CaM to AurA resulted in the appearance of a substantial S 51 or S 53 -phosphorylated AurA species (QRVLCP-S(51)-NSSQR), as well as additional phosphorylation events on S 66 or S 67 , and S 98 . Interestingly, phosphorylation of S 53 of the Xenopus AurA ortholog (analogous to S 51 in human AurA) has been previously shown to be a product of mitotic auto-phosphorylation, and to stabilize AurA from proteasomal degradation at mitotic exit [38] , [39] . Definition of CaM-binding sites on AurA CaM binding is typically modulated by a combination of defined amino acid motifs and a disordered secondary structure with the potential to form an α-helix [40] . We used four programs for predicting intrinsically disordered regions in proteins (IUPRED, MetaPRDOS, PONDR_FIT and VL3) to analyse AurA structure ( Fig. 4a ). This analysis showed that consensus regions encompassed within approximately residues 1–127 and 385–403 were predicted to be disordered. A crystal structure of residues 100–403 of AurA has been determined [37] (Protein Data Bank entry 2J4Z ), and only residues 126–389 are seen in the density map, confirming the disorder prediction. These residues also coincide with the canonical N- and C-terminal kinase domains, for example, as defined by the PFAM database [41] . In addition, we used the secondary structure prediction program PSIPRED [42] , [43] on a set of AurA orthologs from mammals and Xenopus ( Fig. 4b ), identifying two regions of helical propensity in the N-terminal disordered region, consisting of residues 59–82 and 111–127 in the human sequence. The C-terminal disordered region is predicted to be coiled, and not an α-helix or β-sheet. However, just before this region, residues 353–364 and 367–387 are α-helices in the experimental structure. 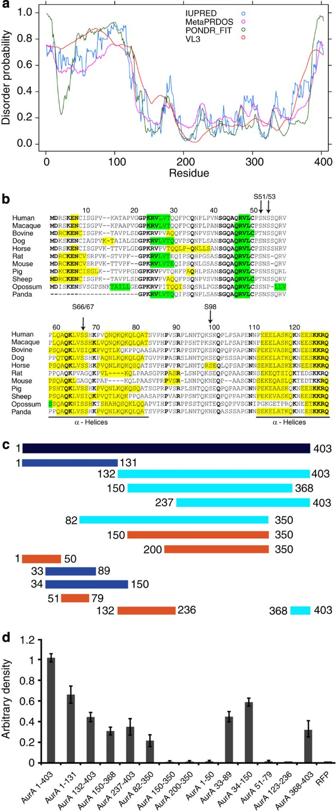Figure 4: Definition of multiple CaM-binding motifs on AurA. (a) Prediction of disordered regions in AurA, using programs IUPRED (blue), MEtaPRDOS (purple), PONDR_FIT (green) and VLE (red). Higher numerical values represent increased likelihood of disorder. (b) Sequence conservation in the AurA amino-terminus (1–127). Predicted β-sheets are shown in green and α-helices in yellow. Arrows indicates Ca2+-dependent AurA auto-phosphorylation sites. Bold represents highly conserved amino acids. (c) Schematic representation of AurA variants used for CaM-binding studies. Intensity of binding is indicated by blue shading, with dark blue indicating the strongest binding, based on data inc. Red indicates no binding. (d) Quantitation of binding of AurA domains with CaM. Graph indicates ratio of coimmunoprecipitated AurA to total AurA, quantified from analysis of blots from three independent experiments in which CaM-Sepharose was used for immunoprecipitation from whole cell lysates expressing red fluorescent protein (RFP), AurA-RFP and RFP-fused domains of AurA, followed by western blotting with antibodies to RFP. Bars indicate standard error. Figure 4: Definition of multiple CaM-binding motifs on AurA. ( a ) Prediction of disordered regions in AurA, using programs IUPRED (blue), MEtaPRDOS (purple), PONDR_FIT (green) and VLE (red). Higher numerical values represent increased likelihood of disorder. ( b ) Sequence conservation in the AurA amino-terminus (1–127). Predicted β-sheets are shown in green and α-helices in yellow. Arrows indicates Ca 2+ -dependent AurA auto-phosphorylation sites. Bold represents highly conserved amino acids. ( c ) Schematic representation of AurA variants used for CaM-binding studies. Intensity of binding is indicated by blue shading, with dark blue indicating the strongest binding, based on data in c . Red indicates no binding. ( d ) Quantitation of binding of AurA domains with CaM. Graph indicates ratio of coimmunoprecipitated AurA to total AurA, quantified from analysis of blots from three independent experiments in which CaM-Sepharose was used for immunoprecipitation from whole cell lysates expressing red fluorescent protein (RFP), AurA-RFP and RFP-fused domains of AurA, followed by western blotting with antibodies to RFP. Bars indicate standard error. Full size image Further refinement of this analysis allowed the mapping of a strong minimal interaction domain to residues 33–89, and suggested weaker binding elements encompassed within residues 82–132, 350–368 and 368–403 ( Fig. 4c,d ). Suggestively, the minimum strong CaM-AurA-binding site encompassed the longest of the predicted α-helices in the N-terminal disordered region (residues 59–82), with the α-helices adjacent to or containing the Ca 2+ -dependent auto-phosphorylation sites (S 51 /S 53 and S 66 /S 67 ). Further, the α-helix, the phosphorylation sites and the flanking sequences show striking conservation through mammals ( Fig. 4b ), implying an important function. The weaker binding of CaM to the other minimal binding elements may be due to unfolding of the protein in some constructs; for example, the predicted helical regions in residues 350–368 are encompassed in the catalytic domain, and would normally be folded. However, we cannot rule out local unfolding of this region and CaM binding in intact AurA, based on interactions of AurA with partner proteins. The work presented here reveals and mechanistically defines a novel role for AurA as a component of rapid calcium signalling responses. In interphase cells, we propose that transient stimuli such as AVP or histamine trigger Ca 2+ release into the cytoplasm, inducing CaM binding and auto-activation of AurA. These activities involve different activation mechanisms than those we have previously reported for AurA in regulation of ciliary disassembly [21] , occurring with much faster kinetics (2-5 min versus 1–2 h) and not influenced by depletion of NEDD9. Although our data do not exclude the possibility that second messengers or cilia-based signalling systems may contribute to the activation of AurA in calcium response, they argue against an essential requirement for such activation. Such transient activation of AurA in response to short-term increases in cytoplasmic calcium may offer a mechanism by which AurA is able to phosphorylate targets such as RalA [20] and microtubules [23] in non-mitotic cells. Interestingly, RalA is itself regulated by Ca 2+ in a non-Ras-dependent activation pathway [44] , and RalA activity has been reported to be controlled by CaM binding [45] . Our data raise the possibility that parallel CaM-dependent activation of AurA may help control the degree and timing of RalA activation in cancer and normal cells. The activation of AurA by Ca 2+ –CaM may also have implications for AurA functions at cilia. The polycystic kidney disease (PKD)-associated genes PKD1 and PKD2 encode cilia-associated, heterodimerizing proteins that function as mechanosensors, internalizing Ca 2+ in response to flow-based cues [46] . This localized release of Ca 2+ may transiently activate AurA, given the proximal location of the AurA protein at the ciliary basal body, allowing AurA to phosphorylate substrates relevant to the mechanosensing process. For example, AurA exists in a stable complex with NEDD9, and NEDD9 (HEF1) has previously been reported to bind the Id2 [47] , a protein that is phosphorylated and influences cell differentiation in response to PKD1/PKD2-mediated signalling [48] . These data also offer insight into control mechanisms operant in the cell cycle-regulated activation of AurA. Dynamic changes in calcium signalling have a key role in meiosis, have been implicated in action at spindle-associated microdomains in mitosis [49] and may also regulate AurA. An attractive feature of Ca 2+ -dependent AurA regulation is that it offers a potential mechanism to help explain the rapid, timed activation of AurA at cell cycle transitions. At present, although multiple proteins have been demonstrated to bind and support AurA activation at the mitotic boundary, most of these also interact with AurA in G2, implying the existence of a triggering event at the actual transition point. The transient increase of cytoplasmic Ca 2+ could provide a suitable mitotic trigger. Such Ca 2+ - and CaM-dependent regulation of the centrosomal proteins centrin and CP110 has been shown to be critical for the action of these proteins in supporting cytokinesis. In this view, Ca 2+ release and CaM binding may be a physiological trigger for AurA during cell cycle, causing conformational changes that are permissive for other AurA-interacting proteins to sustain its activity during long-term rather than transient responses. Intriguingly, calcium signalling differs significantly in cancerous [50] versus normal cells, promoting increased cell proliferation through the abnormal activation of numerous calcium-responsive signalling pathways. Hence, our work also raises the possibility that the enhanced AurA activity often found in tumours may, in part, arise from an abnormal calcium signalling environment. These points merit further investigation. Plasmids and cell culture FLAG- and glutathione S-transferase (GST)-fused HEF1 were expressed from the vectors pCatch-FLAG [51] and pGEX-2T [52] , respectively, as previously described. AurA and derivatives were expressed from pCMV-SPORT6-C6 (OpenBiosystems) and pcDNA3.1-mRFP vectors. A PCR product of mRFP was ligated into pcDNA3.1(+) (Invitrogen) to create pcDNA3.1-mRFP. pcDNA3.1-mRFP was used as a negative control. Catalytically inactive AurA (K162R) was prepared using a site-directed mutagenesis kit (Stratagene). HEK293 cells were maintained in Dulbecco's modified Eagle's medium with 10% fetal bovine serum plus penicillin/streptomycin. The immortalized human kidney proximal tubular cell line (HK-2, ATCC, cat. no. CRL-219) was grown to subconuence in keratinocyte media (Invitrogen). We transiently transfected HEK293 cells with expression constructs for HEF1 and AurA using Lipofectamine and Plus reagent (Invitrogen) according to the manufacturer's instructions. Immunofluorescence Cells growing on coverslips were fixed with 4% paraformaldehyde (10 min) and cold methanol (5 min), permeabilized with 1% Triton X-100 in phosphate-buffered saline (PBS), blocked in 1× PBS with 3% bovine serum albumin and incubated with antibodies using standard protocols. Primary antibodies included mouse anti-AurA (BD Biosciences; 1:200) and rabbit polyclonal anti-phospho-AurA/T288 (Cell Signaling; 1:100). Secondary antibodies labelled with Alexa-488, Alexa-568 and DAPI (4',6-diamidino-2-phenylindole) to stain DNA, were from Molecular Probes/Invitrogen (1:2000). Confocal microscopy was performed using a Nikon C1 spectral confocal microscope (Nikon). Western blotting and immunoprecipitation Recombinant Hexa-histidine AurA was produced in a baculovirus expression system. For western blotting and immunoprecipitation, mammalian cells were disrupted in CelLytic M lysis buffer (Sigma) supplemented with a protease and phosphates inhibitor cocktails (Roche). Whole-cell lysates were used either directly for SDS polyacrylamide gel electrophoresis (SDS–PAGE) or for immunoprecipitation. Immunoprecipitation samples were incubated overnight with antibody at 4 °C, and subsequently incubated for 2 h with protein A/G-sepharose (Pierce), washed and resolved by SDS–PAGE. Western blotting was done using standard procedures, and developed by chemiluminescence using the West-Pico system (Pierce). Primary antibodies included mouse anti-NEDD9 mAb (clone 2G9 [9] ; 1:1000), anti-AurA (BD Biosciences; 1:3000), anti-phospho-AurA-T 288 and anti-GST mAb (Cell Signaling; 1:2000), anti-V1aR (Santa Cruz Biotechnology; 1:600) and anti-β-actin mAb (AC15, Sigma;1:20,000). Polyclonal anti-AurA agarose-immobilized conjugate (Bethyl) were used for immunoprecipitations. Secondary anti-mouse and anti-rabbit horseradish peroxidase-conjugated antibodies (GE Healthcare) were used at a dilution of 1:10,000 for visualization of western blots. Image analysis was done using NIH ImageJ—Image Processing and Analysis software (National Institutes of Health), with signal intensity normalized to β-actin or total AurA level. Structural analysis Four programs that predict intrinsically disordered regions were used via their webservers: IUPRED [53] , MetaPRDOS [54] , PONDR_FIT [55] and VL3 [56] . PSI-BLAST [57] was used to search the Uniprot database [58] to find orthologs of AurA and to identify crystal structures of AurA in the Protein Data Bank. A selection of these sequences was retrieved and a multiple sequence alignment was performed with Clustal W [59] . The program PSIPRED [43] was used to predict secondary structure for these sequences based on single sequence predictions, rather than multiple sequence alignments from PSI-BLAST. CaM association studies Cell lysates in lysis buffer (PBS with 1% Triton X-100) or purified GST fusion protein diluted in binding buffer (50 mM Tris–HCl (pH 7.6), 120 mM NaCl, 1% Brij) were incubated with CaM-Sepharose 4B (GE Healthcare) or control Sepharose for 1–2 h at 4 °C, as indicated in the figure legends. In defined in vitro experiments, AurA was purified from baculovirus, as previously described [21] , whereas recombinant proteins AurB or Src were obtained from Millipore. After washing, beads were boiled in SDS sample buffer and separated by SDS–PAGE followed by western blotting. Phosphorylation assays MBP, histone H3 (Upstate) and histone H1 (Upstate) were used as positive and negative controls for AurA phosphorylation using standard methods. Parallel aliquots without γ- 32 P(ATP) were processed for SDS–PAGE/Coomassie staining (Invitrogen). To assess CaM-dependent AurA activation, in vitro kinase assay was performed using AurA purified from baculovirus or according the protocol described above, in the presence of 1 μM CaM (Calbiochem) and 1 mM Ca 2+ . For kinase assay without Ca 2+ , 1 mM EGTA was substituted for 1 mM Ca 2+ in the kinase buffer. Endogenous phospho-T 288 -AurA protein in HK2 cells was detected by PathScan Phospho-AurA Sandwich ELISA kit (Cell Signaling) according to the manufacturer's instructions. Mass spectrometry After an in vitro kinase reaction with AurA produced from baculovirus in the presence or absence of CaM plus 1 mM CaCl 2 , gels were stained with Coomassie blue and phosphorylated AurA bands were excised and sequenced at the Taplin Biological Mass Spectrometry Facility at Harvard Medical School, by using microcapillary reverse-phase HPLC nanoelectrospray tandem mass spectrometry on a Finnigan LCQ DECA quadrupole ion trap mass spectrometer. Statistical analysis Statistical comparisons were made using a two-tailed Student's t -test. Experimental values were reported as the means ± s.e. Differences in mean values were considered significant at P <0.05. All calculations of statistical significance were made using the GraphPad InStat software package (GraphPad). How to cite this article: Plotnikova, O. V. et al . Rapid calcium-dependent activation of Aurora-A kinase. Nat. Commun. 1:64 doi: 10.1038/ncomms1061 (2010).